Persistent infection with Crohn’s disease-associated adherent-invasiveEscherichia colileads to chronic inflammation and intestinal fibrosis Crohn’s disease is a chronic inflammatory condition of the gastrointestinal tract in which alterations to the bacterial community contribute to disease. Adherent-invasive Escherichia coli are associated with human Crohn’s disease; however, their role in intestinal immunopathology is unclear because of the lack of an animal model compatible with chronic timescales. Here we establish chronic adherent-invasive Escherichia coli infection in streptomycin-treated conventional mice (CD1, DBA/2, C3H, 129e and C57BL/6), enabling the study of host response and immunopathology. Adherent-invasive Escherichia coli induces an active T-helper 17 response, heightened levels of proinflammatory cytokines and fibrotic growth factors, with transmural inflammation and fibrosis. Depletion of CD8+ T cells increases caecal bacterial load, pathology and intestinal fibrosis in C57BL/6 mice, suggesting a protective role. Our findings provide evidence that chronic adherent-invasive Escherichia coli infections result in immunopathology similar to that seen in Crohn’s disease. With this model, research into the host and bacterial genetics associated with adherent-invasive Escherichia coli -induced disease becomes more widely accessible. Rates of inflammatory bowel disease (IBD) in North America remain among the highest in the world, and international data indicate a rising incidence of Crohn’s disease (CD) in many regions, especially among the paediatric and adolescent population [1] , [2] , [3] , [4] . CD pathogenesis is complex and is influenced by genetic and environmental factors and immune-mediated injury to the gut mucosa brought about by prolonged activation of the mucosal immune system [5] , [6] . Genome-wide association studies link ~100 risk loci to CD; however, these susceptibility genes in aggregate account for less than 25% of the predicted heritability in CD [7] , supporting the view that non-genetic factors have an important role in disease emergence. Among these, changes to the composition of the intestinal bacterial community and its interactions with the intestinal barrier confer the majority of risk [8] , [9] . Mounting evidence indicates that the gut microbiota is an active disease modifier, providing antigens that drive chronic inflammatory reactions [10] . Metagenomic and biopsy studies have revealed unique compositions of the gut microbiota in patients with IBD compared with healthy controls [9] , [11] , [12] , suggesting that specific alterations to the gut microbiota could bring about the distinct clinical features of CD. Much experimental and observational data implicate infectious agents in the initiation, maintenance and risk of chronic inflammation in CD [10] , [13] . Escherichia coli is a predominant Gram-negative species in the healthy intestine where it has an important role in gut homeostasis. Through acquisition of virulence factors E. coli can acquire pathogenic traits that participate in intestinal and extraintestinal disease processes [14] . Adherent-invasive E. coli (AIEC) is a mucosa-associated bacterium often found in CD [15] , [16] . AIEC can invade epithelial cells and induce a proinflammatory state, suggesting that they might participate in chronic disease processes that have an immunological basis. Genome sequencing of AIEC by our group and others [17] , [18] , [19] revealed a close relationship between AIEC and extraintestinal pathogenic E. coli , lending support to the view that AIEC represents a family of evolved E. coli lineages that may, in some host niches, be pathogenic in a manner unique from frank enteric pathogens. The predominance of AIEC in human CD patients in conjunction with a growing body of experimental work has generated interest in the role of AIEC in the initiation and/or progression of chronic inflammation in the gut. The prototype AIEC strain, LF82 (ref. 20 ), induces proinflammatory cytokines and inflammation in dextran sulphate sodium (DSS)-treated transgenic mice that express human carcinoembryonic antigen-related cell adhesion molecule (CEACAM) receptors, which are thought to be host cell receptors interacting with LF82 type I pili [21] . However, research into the role of AIEC in promoting CD-like disease has been limited by the lack of a suitable animal model that gives rise to long-term AIEC colonization without the need for coadministration of colitogenic chemicals to transgenic mice [21] . Thus, open questions remain whether AIEC induces the chronic inflammation and fibrosis that is pathognomonic of human CD. To overcome these limitations we have developed a chronic infection model using AIEC strain NRG857c in five conventional mouse strains, where colonization persists for months and is accompanied by chronic transmural inflammation and fibrosis. This new model has several advantages over DSS-treated CEABAC10 mice infected with AIEC strain LF82 (ref. 21 ). First, our model uses widely available conventional mice that are streptomycin-pretreated but without colitogenic chemicals. Second, AIEC infection is chronic with no animal mortality, whereas LF82-infected CEABAC10 mice experience 80% mortality within 7 days [21] . The available genome sequence of NRG857c AIEC offers a ready system to explore microbial determinants of long-term carriage, disease initiation and progression. Using this model, we show that chronic AIEC infection induces chronic inflammation in the gastrointestinal tract and immunopathology in the small and large bowel of mice. This immunological host response involves cytokines, profibrotic mediators and immune cell infiltration, which resemble that seen in human CD. From depletion studies we show that CD8+ lymphocytes, in part, have a role in limiting AIEC propagation and protecting the host from immunopathology. This new model of AIEC-induced intestinal inflammation and fibrosis will enable new understanding of the role of AIEC in chronic gut inflammation, and will help to uncover the bacterial and host genetics underlying pathophysiological processes in CD. Establishing chronic AIEC infection in mice A previous study reported that wild-type mice orally challenged with the AIEC strain LF82 showed neither colonization nor gut inflammation after 7 days [21] . An alternative model using DSS-treated transgenic mice that express human CEACAM receptors (CEABAC10) was developed, showing severe colitis with 80% mortality over 7 days [21] . As CD is a chronic disease in humans, we sought to develop a long-term infection model using mice that are widely available. We pretreated five conventional strains of mice (CD1, DBA/2, 129e, C3H and C57BL/6) with a single dose of streptomycin 24 h before infection with the human AIEC isolate NRG857c that we previously characterized genetically [17] . Our work began by first comparing the ability of the AIEC reference strain (LF82) to colonize conventional mouse strains in competition with NRG857c. When an equal mixture of wild-type LF82 and NRG857c were inoculated into CD1 mice, the LF82 strain was cleared through competitive colonization by ~day 4 post infection ( Fig. 1a ). CD1 mice monocolonized with LF82 had a consistently lower AIEC burden compared with mice infected with NRG857c over 28 days ( Fig. 1b ). This indicated that NRG857c has greater within-host fitness compared with LF82, which focused our attention on the host response to NRG857c. Immunohistochemical (IHC) staining of AIEC in 28 day-infected caecal tissue from CD1 mice confirmed robust colonization, primarily located at the base of intestinal crypts and within mucosal goblet cells ( Fig. 1c ). Time-course experiments over 63 days of AIEC infection showed chronic and generally stable colonization of the ileum, caecum, and colon of CD1, 129e, DBA/2 and C3H mice ( Fig. 2a–d ). The notable difference was that by day 63, the bacterial load had decreased to undetectable levels in C57BL/6 mice in the colon and the caecal and ileal tissues ( Fig. 2e ) but remained stably high in the other four mouse strains tested. We also found very low levels of viable AIEC in the liver and spleen intermittently throughout the experiment in all mice ( Fig. 2a–e ). AIEC infection of C3H mice caused a reduction in size of both colon and caecum, whereas in DBA/2 and C57BL/6 mice atrophy was only seen in the colon and caecum, respectively ( Supplementary Fig. S1 ). These results demonstrate that AIEC NRG857c can chronically colonize the gut of streptomycin-treated conventional mice that lack CEACAM receptors. 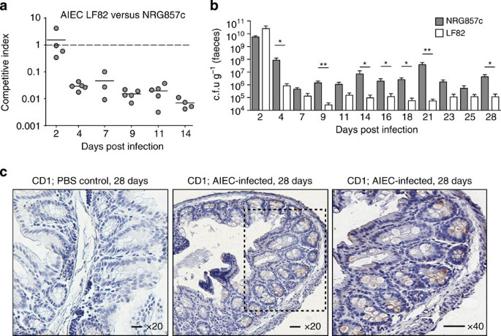Figure 1: Competitive infection between AIEC strain LF82 and NRG857c and NRG857c localization in the caecum of CD1 mice. (a) Mice were infected with an equal mixture of AIEC strains LF82 and NRG857c, and individual AIEC populations were enumerated in faecal output. Each data point represents the competitive index from an individual animal. Solid lines indicate the geometric mean for each group (n=5). (b) Quantification of AIEC in faeces of monocolonized mice. *P<0.05; **P<0.01 (Mann–Whitney’s test). Data are means with s.e. from four to nine mice per group from two experiments. (c) IHC analysis of caecal sections 28 days after infection with NRG857c and in PBS controls. Tissue was fixed and processed for IHC staining using an antibody directed against the O83 antigen found on AIEC strain NRG857c (brown stain in images). Images are representative from two separate experiments. Scale bar, 200 μm. Figure 1: Competitive infection between AIEC strain LF82 and NRG857c and NRG857c localization in the caecum of CD1 mice. ( a ) Mice were infected with an equal mixture of AIEC strains LF82 and NRG857c, and individual AIEC populations were enumerated in faecal output. Each data point represents the competitive index from an individual animal. Solid lines indicate the geometric mean for each group ( n =5). ( b ) Quantification of AIEC in faeces of monocolonized mice. * P <0.05; ** P <0.01 (Mann–Whitney’s test). Data are means with s.e. from four to nine mice per group from two experiments. ( c ) IHC analysis of caecal sections 28 days after infection with NRG857c and in PBS controls. Tissue was fixed and processed for IHC staining using an antibody directed against the O83 antigen found on AIEC strain NRG857c (brown stain in images). Images are representative from two separate experiments. Scale bar, 200 μm. 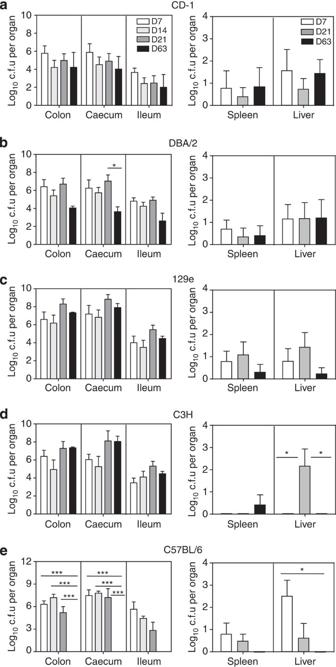Figure 2: Bacterial load of AIEC in various mouse strains. Groups of conventional mice (a) CD1, (b) DBA/2, (c) 129e, (d) C3H and (e) C57BL/6 were infected with AIEC NRG857c and organs were collected following infection. Data are expressed as the means with s.e. of four mice per time point from two independent experiments. *P<0.05, ***P<0.001 (one-way analysis of variance with Tukey’s post test) for comparisons between the time points indicated by bars. Full size image Figure 2: Bacterial load of AIEC in various mouse strains. Groups of conventional mice ( a ) CD1, ( b ) DBA/2, ( c ) 129e, ( d ) C3H and ( e ) C57BL/6 were infected with AIEC NRG857c and organs were collected following infection. Data are expressed as the means with s.e. of four mice per time point from two independent experiments. * P <0.05, *** P <0.001 (one-way analysis of variance with Tukey’s post test) for comparisons between the time points indicated by bars. Full size image Inflammation and pathology during chronic AIEC infection We next investigated whether protracted colonization by AIEC NRG857c was proinflammatory. Histological analyses of haematoxylin and eosin-stained caecal tissue ( Fig. 3 ) and colon ( Supplementary Fig. S2 and S3 ) from all mouse lines were performed at various times after AIEC infection, and the ileal tissue was analysed at 21 days post infection in CD1 and C57BL/6 mice ( Supplementary Fig. S4 ). AIEC-colonized animals exhibited chronic persistent inflammation to varying degrees, depending on the genetic background of the mouse ( Fig. 3a and Supplementary Figs S2–S4 ). AIEC-infected caecum of all mouse strains displayed transmural inflammation and oedema, as well as crypt hyperplasia ( Fig. 3a ). Widespread sloughing of epithelial cells was present with crypt loss in some regions in CD1 and 129e mice (day 7 and 14). Caecum of infected DBA/2, C3H and C57BL/6 mice had submucosal and mucosal ulceration, and thickened mucosa indicative of crypt hyperplasia along with loss of goblet cells. Cellular infiltration was evident in the mucosa, submucosa and lumen. In CD1 mice (day 21), regions of epithelial destruction were replaced by immune cell infiltration, whereas in the other mouse strains epithelial regeneration and repair were apparent by day 21 even though there was continued cellular infiltration. Similar results were seen in infected colons from all mouse lines ( Supplementary Fig. S2 and S3 ), although the pathology scores tended to be lower than that for the caecum. AIEC has been isolated from the ileum of humans with CD and we found consistent AIEC colonization of this site in mice. Therefore, we scored ileal immunopathology 21 days after infection and observed infiltration of cells throughout the villi in the ileal mucosa, epithelial destruction and crypt ulceration in both the mouse lines examined ( Supplementary Fig. S4 ). These data demonstrated that chronic AIEC infection leads to tissue pathology in the small and large bowel, with more extensive pathology seen in the caecum. 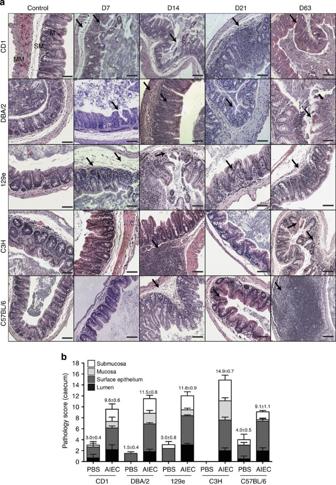Figure 3: Inflammation and tissue pathology in the caecum following chronic infection with AIEC. (a) Haematoxylin and eosin staining of caecal sections from CD1, DBA/2, 129e, C3H and C57BL/6 mice after AIEC infection, and from uninfected controls. Images are representative of two experiments with four mice per time point. MM, muscularis mucosa; SM, submucosa; M, mucosa; L, lumen. Arrows indicate submucosa oedema, desquamation, hyperplasia, inflammatory cellular infiltrates and epithelial sloughing. (b) Caecal pathology was scored 3 weeks after infection. Scores represent an average of five views per section, and data are expressed as the means with s.d. for each group. Original magnification: × 200; scale bar, 200 μm. Figure 3: Inflammation and tissue pathology in the caecum following chronic infection with AIEC. ( a ) Haematoxylin and eosin staining of caecal sections from CD1, DBA/2, 129e, C3H and C57BL/6 mice after AIEC infection, and from uninfected controls. Images are representative of two experiments with four mice per time point. MM, muscularis mucosa; SM, submucosa; M, mucosa; L, lumen. Arrows indicate submucosa oedema, desquamation, hyperplasia, inflammatory cellular infiltrates and epithelial sloughing. ( b ) Caecal pathology was scored 3 weeks after infection. Scores represent an average of five views per section, and data are expressed as the means with s.d. for each group. Original magnification: × 200; scale bar, 200 μm. Full size image AIEC inflammation involves Th1 and Th17 responses The lamina propria of CD lesions contains elevated levels of interferon-γ (IFN-γ) [22] and tumour necrosis factor-α (TNF-α). T-helper 17 (Th17) is also a predominant response in CD through the interleukin (IL)-17/IL-23 axis, which might be involved in the maintenance of transmural intestinal inflammation [6] , [23] , [24] . We tested whether the inflammatory mediators TNF-α, IFN-γ and IL-17 were induced during chronic AIEC infection. We found a significant increase in TNF-α and (to a lesser extent) IFN-γ in the colon and caeca of AIEC-infected CD1 and C57BL/6 mice compared with uninfected controls (day 21) ( Fig. 4a ). TNF-α and IFN-γ levels were not different in the inflamed colon and caecum of DBA/2, 129e and C3H mice compared with that in the uninfected controls. IL-17 was significantly increased in the colon and caeca of all mice, suggesting a Th17 response in our model ( Fig. 4c ). MCP-1 is an important chemokine for recruitment of mononuclear cells to the site of inflammation in IBD and contributes to transmural intestinal fibrosis when overexpressed in the gut [25] . There was a significant increase in MCP-1 expression in the colon and caeca of CD1, DBA/2, C3H and C57BL/6 mice ( Fig. 4d ), with higher levels in the caeca compared with that in the colon, consistent with the pathology. 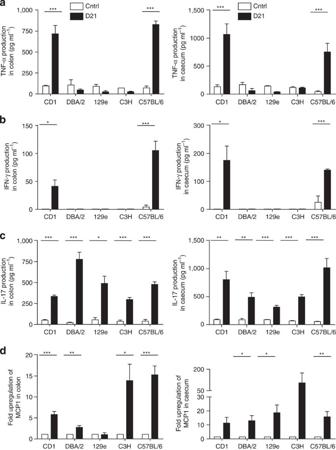Figure 4: Th1 and Th17 inflammatory responses in the colon and caecum following chronic AIEC infection. The colon and caecum from groups of mice were removed and processed. (a) TNF-α, (b) IFN-γ, (c) IL-17 and (d) MCP-1 were measured from the colon (left panels) and caecum (right panels) by enzyme-linked immunosorbent assay. Data are the mean with s.e. from four mice per group and from two independent experiments. *P<0.05, **P<0.01, ***P<0.001 (compared with uninfected controls; one-way ANOVA with Dunnett post test). Ctrl, control. Figure 4: Th1 and Th17 inflammatory responses in the colon and caecum following chronic AIEC infection. The colon and caecum from groups of mice were removed and processed. ( a ) TNF-α, ( b ) IFN-γ, ( c ) IL-17 and ( d ) MCP-1 were measured from the colon (left panels) and caecum (right panels) by enzyme-linked immunosorbent assay. Data are the mean with s.e. from four mice per group and from two independent experiments. * P <0.05, ** P <0.01, *** P <0.001 (compared with uninfected controls; one-way ANOVA with Dunnett post test). Ctrl, control. Full size image Chronic infection with AIEC induces intestinal fibrosis Following AIEC infection, the colon and caecum had a hardened texture as described previously in Salmonella -induced colitis [24] . We investigated whether these observations reflected fibrotic processes by staining tissues with Masson’s trichrome and picrosirius red (PSR) to visualize extracellular matrix (ECM) deposition. Tissues from uninfected control animals had a thin layer of ECM restricted to the submucosal layer of the caecum, whereas caecal tissue from AIEC-infected mice had extensive ECM deposition as early as day 7 with dense fibrosis evident in all mouse strains at later time points ( Fig. 5a–c and Supplementary Fig. S5 ). Matrix deposition was evident in regions with submucosal oedema as well as thin and thick collagen fibrils in the caecal muscularis mucosa. Heavy ECM deposition spreading into the mucosal area interspersed among the inflammatory cells of the lamina propria was evident in DBA/2, CD1 and C57BL/6 mice (day 14) ( Fig. 5a–c ). Fibrosis persisted throughout the entire caecal wall in these mice on day 63 post infection, demonstrating that chronic AIEC infection leads to progressive transmural caecal fibrosis. Colonic fibrosis was less pronounced in all mouse strains, with the general exception being AIEC-infected DBA/2 mice that showed extensive ECM deposition not only in the submucosa and muscularis mucosa but also interspersed throughout the lamina propria inflammatory cells ( Supplementary Figs S6 and S7 ). 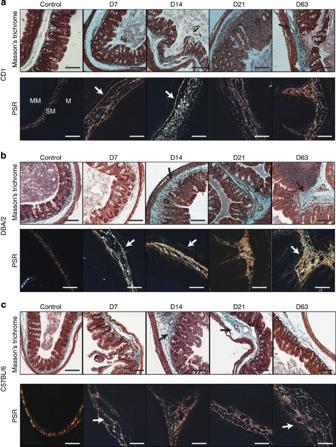Figure 5: Intestinal fibrosis in the caecum following chronic AIEC infection. Masson’s trichrome and PSR staining of caecal tissue from (a) CD1, (b) DBA/2 and (c) C57BL/6 mice following AIEC infection and from uninfected controls. Black arrows in the Masson’s trichrome panels indicate collagen deposition (green) in the submucosa and the mucosa surrounding inflammatory cellular infiltrates. White arrows in the PSR panels indicate collagen fibrils (large collagen fibers, yellow/orange; thinner fibers, green) in the muscularis mucosa, submucosa and mucosa. MM, muscularis mucosa; SM, submucosa; M, mucosa. Images are representative of two experiments with four mice per time point. Original magnification: × 200; scale bar, 200 μm. Figure 5: Intestinal fibrosis in the caecum following chronic AIEC infection. Masson’s trichrome and PSR staining of caecal tissue from ( a ) CD1, ( b ) DBA/2 and ( c ) C57BL/6 mice following AIEC infection and from uninfected controls. Black arrows in the Masson’s trichrome panels indicate collagen deposition (green) in the submucosa and the mucosa surrounding inflammatory cellular infiltrates. White arrows in the PSR panels indicate collagen fibrils (large collagen fibers, yellow/orange; thinner fibers, green) in the muscularis mucosa, submucosa and mucosa. MM, muscularis mucosa; SM, submucosa; M, mucosa. Images are representative of two experiments with four mice per time point. Original magnification: × 200; scale bar, 200 μm. Full size image A number of profibrotic mediators are involved in intestinal fibrosis, including growth factors and the chemokine MCP-1 (refs 24 , 26 , 27 ). Transforming growth factor-β1 (TGF-β1) is believed to be a primary driver of fibrosis and can stimulate other growth factors, including connective tissue growth factor (CTGF), involved in fibroblast proliferation, and insulin-like growth factor (IGF1), all of which are upregulated in fibrotic tissues of CD patients [28] . We measured mRNA levels of these markers by reverse transcriptase–PCR (RT–PCR) in mice infected with AIEC for 21 days. TGF-β1 , CTGF and IGF1 mRNA was higher in the caecum compared with that in the colon of all AIEC-colonized mice ( Fig. 6a–c ). AIEC-infected C57BL/6 mice had higher expression levels of TGF-β1 , CTGF and IGF1 compared with that in the other mouse strains, with a greater contribution in the colon. These data indicated that AIEC infection is associated with increased expression of profibrotic mediators, primarily in the caecum where fibrosis was greatest, and that the mouse genetic background influences the magnitude of the tissue response. Increased deposition of collagen type I and III occurs in intestinal strictures in CD patients. Using quantitative RT–PCR analysis of fibrotic tissue, we found elevated Col1a2 and Col3a1 mRNA in the caeca of all AIEC-colonized mouse strains, with more variable levels in the colon ( Fig. 6d ). Overall, the patterns of cytokines, growth factors, profibrotic mediators and collagen types observed in the caeca and colons of mice during chronic AIEC infection resemble profiles seen in CD patients [10] , [29] . 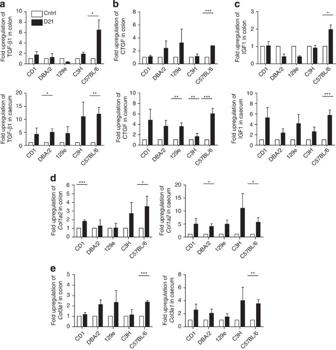Figure 6: Profibrotic mediators associated with AIEC-induced fibrosis. The mRNA levels of (a) TGF-β1, (b) CTGF and (c) IGF1 expression in the colon (upper panels) and caecum (lower panels) was determined 3 weeks post AIEC infection. Data were normalized to 18s RNA and expressed as fold-change relative to the uninfected control. Quantification of (d) collagen type I (Col1a2) and (e) collagen type III (Col3a1) was determined by quantitative RT–PCR. Data were normalized to 18s RNA and expressed as fold-change relative to the uninfected PBS-treated control. Data are expressed as the means with s.e. from four mice per group, representative of two independent experiments. *P<0.05, **P<0.005, ***P<0.001 compared with uninfected PBS-treated controls (one-way analysis of variance with Dunnett’s post test). Figure 6: Profibrotic mediators associated with AIEC-induced fibrosis. The mRNA levels of ( a ) TGF-β1, ( b ) CTGF and ( c ) IGF1 expression in the colon (upper panels) and caecum (lower panels) was determined 3 weeks post AIEC infection. Data were normalized to 18s RNA and expressed as fold-change relative to the uninfected control. Quantification of ( d ) collagen type I ( Col1a2 ) and ( e ) collagen type III ( Col3a1 ) was determined by quantitative RT–PCR. Data were normalized to 18s RNA and expressed as fold-change relative to the uninfected PBS-treated control. Data are expressed as the means with s.e. from four mice per group, representative of two independent experiments. * P <0.05, ** P <0.005, *** P <0.001 compared with uninfected PBS-treated controls (one-way analysis of variance with Dunnett’s post test). Full size image CD8+ lymphocytes have a protective role in C57BL/6 mice Having observed high levels of TNF-α and IL-17 in addition to transmural inflammation and fibrosis in C57BL/6 mice, we examined the immunological response in these mice in greater detail. By IHC analysis, caecal tissue from AIEC-infected C57BL/6 mice showed a marked increase in F4/80-positive cells ( Fig. 7a ), a marker for mature mouse macrophages, elevated infiltration of FoxP3-positive cells ( Fig. 7b ) and greater accumulation of CD3-positive T cells throughout the mucosa ( Fig. 7c ). The increased cytokine and fibrotic responses in AIEC-infected mice was consistent with a Th1/Th17 response. This was particularly evident in C57BL/6 mice that were able to clear AIEC at later time points, yet continued to exhibit a pathophysiological response in the gut typically attributed to T-cell immune responses. Because of the increase in CD3+ cells seen in AIEC-infected mice, we infected Rag1 −/− mice with AIEC, as well as depleted either CD4+ or CD8+ T cells from AIEC-infected C57BL/6 mice using specific antibodies. Compared with mice treated with control IgG, AIEC-infected Rag1 −/− mice and mice depleted of CD8+ cells had a 4–5 log increase in faecal AIEC between days 7 and 21 after infection, whereas CD4-depleted mice has an intermediate phenotype with a 1–3 log increase ( Fig. 8a ). CD8-depleted mice maintained consistently high levels of AIEC even at day 21, accompanied by significantly increased pathology characterized by hyperplasia and high amounts of immune cell perfusion into the intestinal lumen as well as the submucosa. Pathology in CD4-depleted mice was not significantly different than that of IgG control-treated mice ( Fig. 8b ). Fibrosis in CD8-depleted mice involved a higher percentage of the caecum compared with IgG control and CD4 depletions ( Fig. 8d ). Finally, we measured the cytokine response from caecal explants taken from immune-deficient mice infected with AIEC. CD4 and CD8 depletion was associated with decreased TNF-α, IFN-γ and IL-17 compared with IgG controls ( Fig. 8e ), suggesting that these cell populations are at least partially responsible for the cytokine responses observed. Flow cytometric analysis of the CD8+ lymphocyte population isolated from the lamina propria showed that AIEC infection increased the proportion of lamina propria CD8 + CD45.2 + cells compared with uninfected controls ( Fig. 8f ) and doubled the number of CD8 + cells expressing IFN-γ ( Fig. 8g ). These data are consistent with CD8+ cells having a role in limiting AIEC colonization in C57BL/6 mice and protecting tissue against immune-mediated pathology. 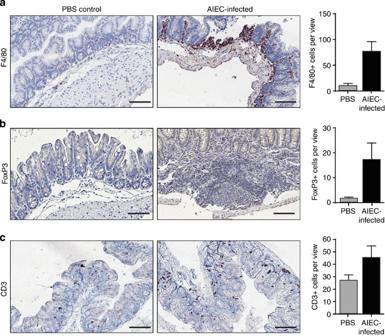Figure 7: Intestinal pathology is associated with increased numbers of immune cells during chronic AIEC infection. Formalin-fixed sections from C57BL/6 mice infected with NRG857c for 21 days were IHC stained for (a) F4/80, (b) Foxp3 and (c) CD3. Each image is representative of three mice per experiment and quantification represent an average of six to eight views per section. Scale bar, 200 μm. Figure 7: Intestinal pathology is associated with increased numbers of immune cells during chronic AIEC infection. Formalin-fixed sections from C57BL/6 mice infected with NRG857c for 21 days were IHC stained for ( a ) F4/80, ( b ) Foxp3 and ( c ) CD3. Each image is representative of three mice per experiment and quantification represent an average of six to eight views per section. Scale bar, 200 μm. 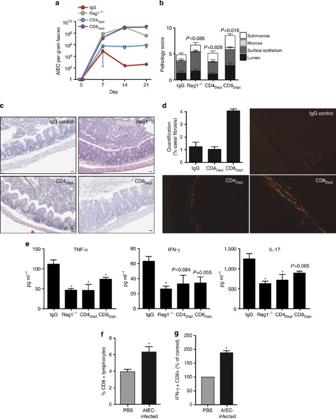Figure 8: CD8+ immune cells are protective role during chronic AIEC infection. (a) Rag1−/−, CD4-, CD8-depleted and IgG control mice were infected with NRG857c (three mice per group, representing two independent experiments). AIEC load in faecal pellets was quantified from immune-depleted mice over time. At day 21, caecal tips were scored for histopathology (b) on haematoxylin and eosin-stained sections (c); scale bar, 50 μm. (d) Caecal sections were stained with PSR for quantification of fibrosis. Original magnification, × 200. (e) Cytokines were measured from caecal explant supernatants by enzyme-linked immunosorbent assay. C57BL/6 mice were infected with NRG857c or mock infected with PBS (three mice per group were pooled and experiment was repeated three times), and at day 21 after infection the caecum was excised and lamina propria immune cells were isolated and stained for FACS analysis. (f) Percentage of CD45.2+ CD8+ lymphocytes measured by flow cytometry of lamina propria cells from AIEC-infected C57BL/6 mice (day 21). (g) The number of CD8+ IFNγ+ lamina propria cells measured by flow cytometry expressed as a percentage of the PBS control. Data are the means with s.e. *P<0.05 (Studentt-test). Full size image Figure 8: CD8+ immune cells are protective role during chronic AIEC infection. ( a ) Rag1 −/− , CD4-, CD8-depleted and IgG control mice were infected with NRG857c (three mice per group, representing two independent experiments). AIEC load in faecal pellets was quantified from immune-depleted mice over time. At day 21, caecal tips were scored for histopathology ( b ) on haematoxylin and eosin-stained sections ( c ); scale bar, 50 μm. ( d ) Caecal sections were stained with PSR for quantification of fibrosis. Original magnification, × 200. ( e ) Cytokines were measured from caecal explant supernatants by enzyme-linked immunosorbent assay. C57BL/6 mice were infected with NRG857c or mock infected with PBS (three mice per group were pooled and experiment was repeated three times), and at day 21 after infection the caecum was excised and lamina propria immune cells were isolated and stained for FACS analysis. ( f ) Percentage of CD45.2+ CD8+ lymphocytes measured by flow cytometry of lamina propria cells from AIEC-infected C57BL/6 mice (day 21). ( g ) The number of CD8+ IFNγ+ lamina propria cells measured by flow cytometry expressed as a percentage of the PBS control. Data are the means with s.e. * P <0.05 (Student t -test). Full size image There is mounting evidence for a microbial aetiology in IBD where the interplay of host genetics and bacterial factors can perpetuate chronic immune activation and profibrotic processes over time. Characterizing the dysbiosis accompanying human CD is underway [10] , [30] , [31] . However, insight into the connection between host genetics, immunology and potentially deleterious microbes in the gut system is in its infancy. AIEC is an E. coli pathotype found with a greater prevalence in the gastrointestinal tract of individuals with CD. We previously conducted a genome-wide comparison between two AIEC isolates; strain NRG857c and the de facto reference strain, LF82 (ref. 17 ). Emerging from this analysis was a clear evolutionary strain relationship, a phylogenic association of AIEC to extraintestinal pathogenic E. coli , and a collection of strain-specific genetic elements encoded on the chromosome and on a large extrachromosomal plasmid unique to each isolate. Previous work in developing a rodent model for AIEC infection showed that LF82 did not colonize conventional mice beyond day 7 following streptomycin treatment and did not elicit intestinal inflammation in the absence of an antecedent DSS treatment [21] , [32] . DSS-treated transgenic mice expressing human CEACAM receptors develop inflammation following LF82 infection, but this treatment is fatal by 1 week in 80% of animals [21] . We showed that AIEC strain NRG857c induces a persistent infection following a single orogastrically delivered dose into five streptomycin-treated conventional mouse lines. AIEC was primarily localized to the crypts in the mucosa and in goblet cells, consistent with its known invasive properties. Infection with NRG857c induced chronic inflammation in the gut with more pronounced immunopathology in the caecum. We found inflammation in the large bowel to be discontinuous, consistent with that seen in CD—itself a disease of discontinuous inflammation. We observed that AIEC colonization persisted in four out of five mouse strains, with the exception being C57BL/6 mice where AIEC levels dropped below our limit of detection by day 63. However, inflammation and pathology persisted (or was not resolved) even when the AIEC level was below detection. Conventional mice are generally tolerogenic towards commensal microbes, but this can be disrupted following engineered genetic deficiencies, spontaneous mutations or perturbations to the microbial composition in the gut [29] . Given these data, it is possible that the chronic inflammation accompanying a persistent AIEC infection could have a lasting imprint on the gut microbial community in favour of a more colitogenic profile. This, in turn, could facilitate continued immune-mediated intestinal injury even after the infectious insult has been diminished or removed. The major cytokines in CD originate from Th1 and Th17 T cells [6] . The inflammation we observed in the mice was associated with high levels of TNF-α and IL-17, and to a lesser extent with IFNγ, all of which decreased following depletion of CD4+ or CD8+ populations. Another study characterizing trinitrobenzene sulphonic acid-induced colitis found no significant change in IFN-γ levels at later time points [27] , suggesting that TNF-α/IFN-γ may be involved earlier in the induction stage. In keeping with this view, a number of inflammatory stages were noted in trinitrobenzene sulphonic acid-induced colitis, including an early Th1-dominant process involving IFN-γ and IL-12p70 that peaked after 1 week. This was succeeded by a gradually increasing Th17 response mediated by IL-17/IL-23 that was maximal by ~8 weeks [33] . The recruitment of CD8+ cells during AIEC infection correlated with some level of control of AIEC in C57BL/6 mice and with decreased pathological response in the tissue. Others have also reported a protective role for CD8+ cells, where CD8+ TCRγδ+ intraepithelial lymphocytes (IELs) aid in clearance of Salmonella infections through eradication of infected epithelial cells [34] . This population of CD8+ IELs was also protective during Listeria monocytogenes infection, as they are capable of inducing bacterial antigen-specific CD8+ T-cell cytotoxic responses [35] . Given the invasive properties of AIEC, CD8+ cells may be a particularly important host cell response to colonization by this organism. We observed elevated numbers of F4/80+ cells and FoxP3+ cells in the caecum of AIEC-colonized mice, the latter of which were virtually absent from AIEC-naive mice. Mucosal FoxP3+ T regulatory cells and activated macrophages are also elevated in paediatric and adult CD [36] , which seems to be a response specific to CD and not ulcerative colitis [37] . TGF-β regulates the development of FoxP3+ cells in CD that correlates with response to anti-TNF infliximab therapy [38] . Therefore, the high TGF-β response of AIEC-infected C57BL/6 mice might be involved in both the fibrotic processes and immune cell recruitment we observed in the mucosa. Future work is required to determine what subset of CD8+ immune cells are providing the protective effect during chronic AIEC infections, and whether it is a combination of both regulatory and cytotoxic CD8+ T cells, and IELs. Progressive inflammation in CD leads to fibrogenic alterations to the ECM that are distinct from ulcerative colitis, which lacks a CTGF and IGF1 response, and does not generally progress to fibrostenotic disease. The histological processes seen in our model resemble active remodelling and fibrosis typical of human CD and other experimental systems [24] , [27] , [39] . Intestinal strictures resected from patients with CD have increased total collagen content [39] , [40] , [41] . Although we did not observe intestinal stricturing, we did observe transmural inflammation as well as upregulated expression of profibrotic growth factors and collagen. The differences in the timing, magnitude and location of intestinal inflammation and fibrosis seen in the various mouse strains might relate to genetically imprinted host susceptibilities that are now tractable in future work. The conventional mouse lines used in our study should facilitate accelerated investigation into the biological mechanisms underlying AIEC-induced colitis and fibrotic disease. Ethics statement All animal experiments were conducted according to guidelines set by the Canadian Council on Animal Care using protocols approved by the Animal Review Ethics Board at McMaster University. Bacterial strains AIEC strain NRG857c (O83:H1) was isolated from an ileal tissue biopsy from a CD patient in Charite Hospital (Berlin, Germany), and its genome has been sequenced and subjected to comparative genomic analysis [17] . NRG857c was cultured in Luria broth (LB) containing chloramphenicol (34 μg ml −1 ) and ampicillin (100 μg ml −1 ). AIEC strain LF82 is the AIEC reference strain used in almost all AIEC literature to date [20] . LF82 was obtained from Alfredo Torres (University of Texas Medical Branch, Galveston, TX) [42] and was cultured in LB broth containing ampicillin (100 μg ml −1 ). Before animal infection, bacteria from overnight cultures were washed, diluted and resuspended in PBS. Animal infections Eight- to ten-week-old female CD1, DBA/2, 129e, C3H and C57BL/6 mice were purchased from Charles River Laboratories. Rag1 −/− mice were purchased from Jackson Laboratories. Animals were housed in a specific pathogen-free barrier facility under Level 2 conditions. Female mice were given 20 mg of streptomycin orally 24 h before infection with 2 × 10 9 colony forming units (c.f.u.) of AIEC NRG857c. Control groups received sterile PBS. For competitive infections, mice were treated as above and infected with a 1:1 ratio (1 × 10 9 c.f.u. each) of wild-type NRG857c and LF82. Following infection, the number of bacteria was monitored in faecal output. To differentiate NRG857c and LF82 in the output pool we took advantage of the different antibiotic resistance profiles of these strains. Faecal homogenates were first plated on LB agar containing 200 μg ml −1 ampicillin and incubated at 37 °C overnight. Colonies were then replica-plated onto LB (no antibiotics) and LB containing ampicillin (200 μg ml −1 ) and chloramphenicol (34 μg ml −1 ) to select for NRG857c. The competitive index was calculated as: (c.f.u. LF82 output /c.f.u. NRG857c output )/(c.f.u. LF82 input /c.f.u. NRG857c input ). AIEC enumeration in tissues Colon, caecum, spleen and liver were collected into cold PBS at necropsy and homogenized using a Mixer Mill. Tissue homogenates were serially diluted and plated on LB agar containing chloramphenicol and ampicillin to select for AIEC NRG857c. After 24 h of incubation at 37 °C, colonies were counted and expressed as c.f.u. per organ. Histopathological evaluation and IHC analysis Mouse colon and caecum were excised at various times after AIEC infection, fixed in buffered 10% formalin, paraffin-embedded, sectioned into 5-μm slices and then stained with haematoxylin and eosin, Masson’s trichrome or PSR by the Histology Services at the McMaster University. Multiple sections from the same tissue from several animals at each time point were scored according to criteria and descriptions previously defined [43] and summarized in Supplementary Table S1 . In some experiments, quantitative analysis of the PSR-stained images taken under polarized light was performed using an ImageJ macro-based algorithm as previously described [44] . IHC staining of formalin-fixed tissue sections was performed using antibodies against F4/80 (1:600) and CD3 (1:1,000) at the Histology Services (McMaster University) and FoxP3+ (1:2000) and O83+ (1:500) staining was done at the Vertex Pharmaceuticals Core Histology Laboratory (Cambridge MA). For O83 antigen staining, caecal sections were taken 28 days post AIEC NRG857c infection and stained with rabbit anti-O83 antibody, and were viewed under bright-field microscopy. IHC quantification represents an average of six to eight views per section with a total of three formalin-fixed sections per mouse group. Cytokine quantification Colon and caecum were removed and washed with cRPMI (10% fetal bovine serum, 1% L -glutamine and 50 μg ml −1 gentamicin). Tissues were cut into pieces, placed in 1 ml of cRPMI and incubated overnight at 37 °C, 5% CO 2 . Levels of TNF-α, IFN-γ and IL-17 were determined using Quantikine murine ELISA kits from R&D systems (Minneapolis, MN) according to the manufacturer’s protocol. mRNA assessment by real-time quantitative PCR Total RNA was extracted from colonic and caecal tissue using TRIzol (Invitrogen). Complementary DNA for RT–PCR was prepared using cDNA SuperMix (Quanta Biosciences). Quantitative PCR was performed with SYBR green SuperMix (Quanta Biosciences) on a Lightcycler 480 (Roche). The primers used are listed in Supplementary Table S2 . The cycling conditions were 95 °C for 5 min and 50 cycles of 95 °C for 10 s, 55 °C for 30 s and 72 °C for 20 s. Data analysis was performed using Lightcycler software v. 1.5. Gene expression was normalized to 18S rRNA and was expressed relative to the uninfected control. In vivo depletion studies Before infection, mice were injected intraperitoneally with 100 μg anti-CD4 (GK1.5) or anti-CD8 (2.43) on day −2, and −1. Injections were repeated on day 1 post infection, and then every 7 days. Isotype control IgG was administered to control mice. Depletion of T cells was confirmed by flow cytometry using an LSR-II (BD Biosciences) then analysed with FlowJo software (Tree Star, Inc.). Isolation and staining of lamina propria immune cells The caecum of infected mice was excised, washed with ice-cold PBS, cut into 5- to 10-mm sections and incubated in PBS, 5% FCS and 5 mM EDTA in a 37 °C orbital shaker for 20 min. Caecal pieces were isolated and then reincubated in fresh PBS/FCS/EDTA buffer for 1 h under previous conditions. Tissue was then digested for two 20-min periods in digestion media (IMEM media (Gibco), 1% HEPES, 0.6 mg ml −1 DNase I (Sigma) and 0.5 mg ml −1 Collagenase VIII (Sigma)) in a 37 °C orbital shaker. After each 20-min digestion, samples were filtered through a 40-μm cell strainer, flow through was collected and placed on ice, and the remaining tissue was reincubated in fresh digestion media. All flow through was combined from digestion incubations, washed and layered over an osmotic 100/30% Percoll (GE Healthcare) gradient. Percoll gradients were centrifuged at 670 g for 30 min at room temperature. Cells from the 100/30% interphase were collected, washed, enumerated and then plated at 1 × 10 6 cells per ml in stimulation media (RPMI, 10% FCS, 1% Pen/Strep, 1% HEPES, 1% non-essential amino acids, 1% L -glutamine (Gibco) with 5 ng ml −1 PMA (Sigma) and 1 μM ionomycin (Sigma)) and incubated at 37 °C, 5% CO 2 for 4 h. GolgiPlug (BD Biosciences) was added to each sample according to the manufacturer’s protocol. Flow cytometric analysis Stimulated cells were isolated and resuspended in ice-cold FACS buffer (PBS, 0.2% BSA). Cells were first incubated with anti-CD16/32 (eBiosciences) antibody for 15 min on ice, then incubated with a combination of anti-CD45.2-Alexa 700 (eBiosciences), anti-CD4-PerCP (BD Biosciences), anti-CD8-PECy7 (eBiosciences) and corresponding controls for 30 min on ice. For intracellular staining, cells were fixed and permeabilized using GolgiPlug Perm/Fix Kit (BD Biosciences) according to the manufacturer’s protocol, and then stained with anti-IFNγ-APC (eBiosciences) or corresponding control. All cells were thoroughly washed after each step. Stained cells were resuspended in FACS buffer and run on an LSR-II flow cytometer (BD Biosciences), then analysed with FlowJo software (Tree Star, Inc.). Statistical analysis Student’s t -test or one-way analysis of variance with Tukey’s or Dunnett’s post test was performed using a 95% confidence interval. All analyses were performed using Graph Prism 4.0 (GraphPad Software Inc., San Diego, CA). A P -value of 0.05 or less was considered significant. How to cite this article: Small, C. L. et al. Persistent infection with Crohn’s disease-associated adherent-invasive Escherichia coli leads to chronic inflammation and intestinal fibrosis. Nat. Commun. 4:1957 doi: 10.1038/ncomms2957 (2013).